Rhythmic actomyosin-driven contractions induced by sperm entry predict mammalian embryo viability Fertilization-induced cytoplasmic flows are a conserved feature of eggs in many species. However, until now the importance of cytoplasmic flows for the development of mammalian embryos has been unknown. Here, by combining a rapid imaging of the freshly fertilized mouse egg with advanced image analysis based on particle image velocimetry, we show that fertilization induces rhythmical cytoplasmic movements that coincide with pulsations of the protrusion forming above the sperm head. We find that these movements are caused by contractions of the actomyosin cytoskeleton triggered by Ca 2+ oscillations induced by fertilization. Most importantly, the relationship between the movements and the events of egg activation makes it possible to use the movements alone to predict developmental potential of the zygote. In conclusion, this method offers, thus far, the earliest and fastest, non-invasive way to predict the viability of eggs fertilized in vitro and therefore can potentially improve greatly the prospects for IVF treatment. In many organisms, cytoplasmic movements triggered by sperm entry are well described. In sea urchins, ascidians and frogs, for example, they are known to be associated with successful progress of developmental events, such as the establishment of embryo polarity [1] , [2] , [3] , [4] , [5] , [6] . However, the nature, mechanism or consequences of cytoplasmic movements caused by sperm entry into the mammalian egg are currently unknown. In mammalian zygotes, sperm entry is linked with reorganization of the cytoskeleton, cortical granules [7] , endoplasmic reticulum [8] and mitochondria [9] . Mammalian fertilization also triggers oscillations of free cytoplasmic Ca 2+ between completion of meiosis and entry into interphase of the first embryonic cell cycle [10] , [11] . Such oscillations regulate not only events immediately following fertilization [12] , [13] , [14] , [15] but were also reported to affect some aspects of subsequent development [13] , [16] , [17] , [18] . Finally, sperm entry also causes changes in zygote shape: formation of the second polar body (PB); protrusion of the fertilization cone (FC) above sperm chromatin [19] , [20] ; and flattening of the zygote along the axis that bisects the FC [21] . Some cytoplasmic motions have been detected in the fertilized mouse egg [22] , yet, the mechanism behind these motions, their relationship to shape changes, and, most importantly, whether they are associated with developmental success have all remained unknown. Here, we first characterize cytoplasmic movements triggered by sperm entry into the mouse egg to describe their relationship with Ca 2+ oscillations, dynamics of zygote shape and cytoskeleton function. We then examine whether the dynamics of these movements can be used to predict developmental success. Combining rapid time-lapse imaging of mouse eggs commencing straight after their fertilization with advanced image analysis based on particle image velocimetry (PIV), reveals previously unnoticed oscillatory changes in the zygote shape on sperm entry. We find that these rhythmic oscillatory changes are accompanied by abrupt actomyosin-dependent cytoplasmic movements that are synchronous with and depend on Ca 2+ oscillations. The calcium transients alone, however, are insufficient for generating cytoplasmic movements as they depend on the incoming sperm and an unexpected pulsation of the FC. Importantly, we find that the characteristics of these movements provide a novel and, thus far, the earliest and quickest non-invasive means of assessing an embryo's quality. We discuss the promise of using such movements to predict an embryo's developmental potential in assisted reproduction clinics. Sperm entry in mouse triggers rhythmic cytoplasmic motions To characterize cytoplasmic movements on fertilization of the mouse egg and to evaluate whether, and if so, how, they relate to other events associated with fertilization, we first filmed eggs from the time immediately after fertilization until pronuclei formation. We then used advanced image analysis based on the PIV method [23] , [24] , [25] , [26] to analyse and quantify these movements ( Fig. 1a ). This revealed that fertilization of the mouse egg was followed by dramatic periodic increases and decreases in velocity of the cytoplasmic movements (that we termed speed peaks; Fig. 1b–d , n =55 unfertilized oocytes and n =125 eggs fertilized in vivo ). This sequence of fast repetitive movements throughout the egg cytoplasm lasted for approximately 4 h, until pronuclei formed. The speed peaks were initially of relatively low amplitude (between anaphase of meiosis II and early FC outgrowth; Stage 1) but subsequently developed significantly greater amplitudes when the FC fully extended (Stage 2). Finally, their amplitude decreased during and following FC regression (Stage 3) ( Fig. 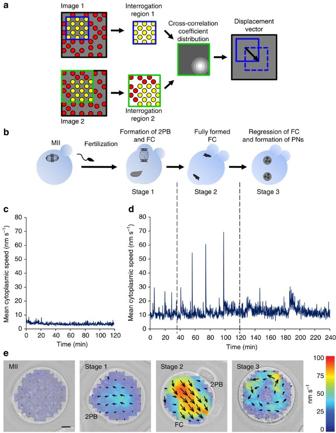Figure 1: Oscillations of cytoplasmic speed in fertilized mouse eggs. (a) Schematic of the cross-correlation image analysis algorithm used to measure the movement of the cell cytoplasm (detailed description in Methods). (b) A schematic representation of the analysed stages: MII: unfertilized eggs in metaphase of the second meiotic division. Stage 1: 2PB is formed and FC first appears. Stage 2: FC is fully formed. Stage 3: FC regresses and pronuclei are formed. (c) Mean cytoplasmic speed in a representative unfertilized egg. (d) Mean cytoplasmic speed in a representativein vivofertilized zygote during Stages 1–3. (e) DIC images with vector patterns representative for unfertilized eggs (MII) and for zygotes in Stage 1–3. For clarity, only every second vector is shown. Length of the vectors and colour of the background indicate speed of the local cytoplasmic movement. Scale bar, 10 μm. 1b,d ; Table 1 ; Supplementary Movie 1 ). In Stage 2, the rapid cytoplasmic movements were greatest in the plane bisecting the FC equatorially and became slower in the more peripheral planes ( Supplementary Fig. S1 ). The PIV analysis revealed that each speed peak was followed by after-movements that usually persisted for more than 4 min and were of lower amplitude. Movements during Stage 3 were exceptions to this rule in that the speed peaks were often less distinct than the after-movements ( Fig. 1d ; Table 1 ). Moreover, we noticed that fertilization led to greater than twofold increase in the basal mean cytoplasmic speed (the speed during interpeak intervals or after the last recorded peak) in comparison to the resting level of unfertilized oocytes ( Fig. 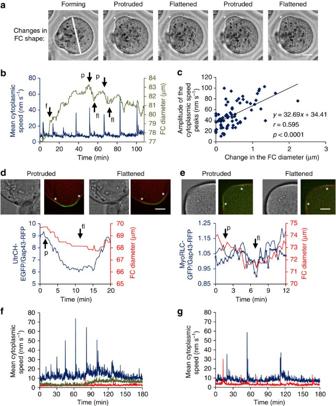Figure 2: Cytoplasmic speed peaks depend on changes in the actomyosin cytoskeleton in the FC region. (a) DIC images of the zygote with a pulsating FC: the FC (marked with an asterisk) protrudes and flattens in a repetitive way. Scale bar, 20 μm. (b) Peaks of the mean cytoplasmic speed in the fertilized mouse egg (blue) correlate with the beginning of a decrease in the FC diameter (green). The FC diameter was measured as shown in (a) from the point of maximum symmetry on the edge of the FC to the other edge of the cell. (c) Change in the FC diameter (measured as a difference between FC diameter immediately before the speed peak and at the timepoint when the speed peak reaches its maximum) correlates with the amplitude of the accompanying speed peak. The Pearson correlation coefficient calculated for these measurements is 0.595 and is statistically significant (P<0.0001). (d) Intensity of UtrCH–EGFP fluorescence in the cortex of the FC (blue) fluctuates as the FC changes its shape (as shown by changes in the FC diameter (red)). Intensity values are presented as a ratio between UtrCH–EGFP and Gap43–RFP (a membrane protein) fluorescence, to eliminate intensity changes caused by shifts in the focus (seeMethodsfor the details). Asterisks show ends of the cortical region in which intensities of UtrCH–EGFP and Gap43–RFP were measured. Scale bar 10 μm. (e) Intensity of MyoRLC–GFP fluorescence in the lower and upper shoulder of the FC (blue line and blue line with crosses, respectively) fluctuates as the FC changes its shape (as shown by changes in the FC diameter (red)). Intensity values are presented as a ratio between UtrCH–EGFP and Gap43–RFP fluorescence. Asterisks mark the regions in which intensities of MyoRLC–GFP and Gap43–RFP were measured. Scale bar 10 μm. (f) Mean cytoplasmic speed in representative zygotes treated with nocodazole (blue line), cytochalasin D (red line) and ML-7 (green line). (g) Mean cytoplasmic speed in representative zygotes treated with taxol (blue line) and jasplakinolide (red line). The peak visible at approx. 90 min is due to a shift in focus. 1c,d ; Table 2 ; Supplementary Movies 1 and 2 ). Figure 1: Oscillations of cytoplasmic speed in fertilized mouse eggs. ( a ) Schematic of the cross-correlation image analysis algorithm used to measure the movement of the cell cytoplasm (detailed description in Methods). ( b ) A schematic representation of the analysed stages: MII: unfertilized eggs in metaphase of the second meiotic division. Stage 1: 2PB is formed and FC first appears. Stage 2: FC is fully formed. Stage 3: FC regresses and pronuclei are formed. ( c ) Mean cytoplasmic speed in a representative unfertilized egg. ( d ) Mean cytoplasmic speed in a representative in vivo fertilized zygote during Stages 1–3. ( e ) DIC images with vector patterns representative for unfertilized eggs (MII) and for zygotes in Stage 1–3. For clarity, only every second vector is shown. Length of the vectors and colour of the background indicate speed of the local cytoplasmic movement. Scale bar, 10 μm. Full size image Table 1 Mean amplitudes of speed peaks and after-movements in control and inhibitor-treated zygotes. Full size table Table 2 Influence of Ca 2+ chelation and cytoskeleton inhibitors and on basal cytoplasmic speed in fertilized mouse eggs. Full size table Our analysis revealed that during Stage 1, the vectors of these abrupt cytoplasmic movements tended to be towards the developing second PB (17/25 speed peaks, 11 zygotes). This directionality changed during Stage 2 such that the vectors were directed towards the FC or sometimes slightly displaced towards the second PB (64/65 speed peaks, 19 zygotes). There was no persisting pattern during the low magnitude after-movements or interpeak intervals in either of these stages. At Stage 3, directionality or any pattern of the speed peaks was not any longer apparent ( Fig. 1e ; Supplementary Table S1 ). These speed peaks ceased after FC regression when pronuclei were observed in the majority of zygotes (49/63, 77.8%) ( Fig. 1d ). Thus, our results indicate that fertilization of the mouse egg triggers speed peaks of cytoplasmic movements that at their strongest are directed towards the FC, forming above the site of sperm entry. Speed peaks rely on actomyosin cytoskeleton and FC pulsations As the direction of the abrupt movements at Stage 2 suggested that the FC could be involved in their generation, we next examined the morphology of the FC throughout this period (69 speed peaks, 14 zygotes). This showed that at each speed peak, the apex of the FC sank inwards and the region where the FC merged into the convex outline of the zygote widened. As a consequence, the diameter of the zygote along the axis of the FC (hereafter called the 'FC diameter') decreased by 1.28±0.66 μm (1.55±0.79% of its length) ( Fig. 2a,b ). The shape of the FC was restored during the interpeak interval ( Fig. 2a ). Interestingly, the extent of reduction of the FC diameter showed a linear association with speed peak amplitude (19 zygotes, 71 speed peaks analysed) ( Fig. 2c ). Figure 2: Cytoplasmic speed peaks depend on changes in the actomyosin cytoskeleton in the FC region. ( a ) DIC images of the zygote with a pulsating FC: the FC (marked with an asterisk) protrudes and flattens in a repetitive way. Scale bar, 20 μm. ( b ) Peaks of the mean cytoplasmic speed in the fertilized mouse egg (blue) correlate with the beginning of a decrease in the FC diameter (green). The FC diameter was measured as shown in ( a ) from the point of maximum symmetry on the edge of the FC to the other edge of the cell. ( c ) Change in the FC diameter (measured as a difference between FC diameter immediately before the speed peak and at the timepoint when the speed peak reaches its maximum) correlates with the amplitude of the accompanying speed peak. The Pearson correlation coefficient calculated for these measurements is 0.595 and is statistically significant ( P <0.0001). ( d ) Intensity of UtrCH–EGFP fluorescence in the cortex of the FC (blue) fluctuates as the FC changes its shape (as shown by changes in the FC diameter (red)). Intensity values are presented as a ratio between UtrCH–EGFP and Gap43–RFP (a membrane protein) fluorescence, to eliminate intensity changes caused by shifts in the focus (see Methods for the details). Asterisks show ends of the cortical region in which intensities of UtrCH–EGFP and Gap43–RFP were measured. Scale bar 10 μm. ( e ) Intensity of MyoRLC–GFP fluorescence in the lower and upper shoulder of the FC (blue line and blue line with crosses, respectively) fluctuates as the FC changes its shape (as shown by changes in the FC diameter (red)). Intensity values are presented as a ratio between UtrCH–EGFP and Gap43–RFP fluorescence. Asterisks mark the regions in which intensities of MyoRLC–GFP and Gap43–RFP were measured. Scale bar 10 μm. ( f ) Mean cytoplasmic speed in representative zygotes treated with nocodazole (blue line), cytochalasin D (red line) and ML-7 (green line). ( g ) Mean cytoplasmic speed in representative zygotes treated with taxol (blue line) and jasplakinolide (red line). The peak visible at approx. 90 min is due to a shift in focus. Full size image Because the actomyosin cytoskeleton is enriched in the FC region [19] , [27] , we considered that this might be responsible for FC pulsations. To evaluate this possibility, we visualized actomyosin throughout these pulsations by injecting oocytes with messenger RNAs encoding either the actin-binding domain of utrophin tagged with EGFP (UtrCH–EGFP [28] ) or the regulatory light chain of myosin II tagged with GFP (MyoRLC–GFP [29] ). Measurements of the mean fluorescence intensity of UtrCH–EGFP in such oocytes, after their fertilization, revealed oscillatory changes in the continuous actin layer underlying the FC; the fluorescence intensity of the actin marker decreased as the FC relaxed and increased as the FC was gradually protruding ( Fig. 2d ; Supplementary Fig. S2 ). Similar results were obtained for the mean fluorescence intensity of MyoRLC–GFP underlying the FC shoulders ( Fig. 2e ; Supplementary Fig. S3 ). Such fluctuations in UtrCH–EGFP and MyoRLC–GFP fluorescence might reflect a change in the amount of the actomyosin in that region. However, as these changes are relatively small, transient and repetitive, it is more likely that they represent contractility of actomyosin encircling the FC leading to its pulsations. As FC movements occurred in time with the cytoplasmic speed peaks directed towards the FC, we next examined whether the actomyosin cytoskeleton was responsible for both. To this end, we used selective inhibitors to interfere with both the actomyosin and microtubule cytoskeletons. Their specificity was confirmed by immunostaining ( Supplementary Fig. S4 ) and their effect on cell cycle progression is presented in Supplementary Table S2 . We found that neither nocodazole-induced depolymerization nor taxol-induced stabilization of microtubules inhibited speed peaks, although their dynamics were slightly changed. Nocodazole treatment increased cytoplasmic speed in some after-movements and in all intervals between speed peaks ( n =38, Fig. 2f ; Tables 1 and 2 ), whereas taxol treatment decreased the amplitude of some speed peaks and after-movements, and cytoplasmic speed in all interpeak intervals ( n =27, Fig. 2g ; Tables 1 and 2 ). In contrast, actin depolymerization with cytochalasin-D or stabilization of actin filaments with jasplakinolide resulted in an almost threefold decrease in basal speed ( Fig. 2f,g ; Table 2 ). Moreover, cytochalasin-D treatment dramatically abolished speed peaks ( Fig. 2f ). Only in 2 out of 21 analysed zygotes (9.5%) were unfocused, low-amplitude speed peaks recorded. Speed peaks were still present in jasplakinolide-treated zygotes ( n =60), although their amplitudes were significantly lower than in controls, and after-movements were virtually undetectable ( Fig. 2g ; Table 1 ). In almost all zygotes, treatment with ML-7, a myosin light chain kinase (MLCK) inhibitor, also blocked cytoplasmic speed oscillations (16/17 zygotes, 94.1%) ( Fig. 2f ), and only a single exceptional zygote showed indistinct low amplitude speed peaks. These experiments also showed that depolymerization or stabilization of microtubules, by respective treatments with nocodazole or taxol, had no effect on either formation and/or maintenance of the FCs. By contrast, FCs did not form in the majority (20/21, 95%) of zygotes treated with cytochalasin-D in agreement with previous studies [13] . Stabilization of actin filaments in zygotes treated with jasplakinolide still permitted formation and/or maintenance of FCs, but they were not as prominent as in controls. FCs were present in just over half of embryos (10/17, 58.8%), when MLCK activity was inhibited and when present, they were less well developed. This accords with the previous conclusion that MLCK activity is involved in formation and maintenance of the FC [27] , [30] . Together, these results indicate that both the cytoplasmic oscillations and FC pulsations depend primarily on the actomyosin cytoskeleton. Cytoplasmic movements depend on Ca 2+ transients As fertilization is known to initiate oscillations of free Ca 2+ (refs 11 , 31 ), we next wished to address whether the actomyosin-mediated speed peaks might depend on these Ca 2+ pulses. To this end, we loaded fertilized eggs with the Ca 2+ -sensitive fluorescent dye FuraRed, and simultaneously collected FuraRed fluorescence and differential interference contrast (DIC) images. In 32 zygotes, all 121 speed peaks were accompanied by an increase in Ca 2+ . The cytoplasmic speed increased exactly (within the resolution of our recording interval) as Ca 2+ levels peaked ( Fig. 3a ; Supplementary Movie 1 ). Only in a single zygote with unusually frequent Ca 2+ oscillations were some Ca 2+ spikes (4/17) not mirrored by speed peaks. In some eggs fertilized by intracytoplasmic sperm injection (ICSI), we managed to record speed peaks accompanying the first Ca 2+ transient. They were of higher amplitude than the rest of Stage 1 speed peaks ( Supplementary Fig. S1 ) corresponding to the first Ca 2+ transient being bigger than subsequent ones. 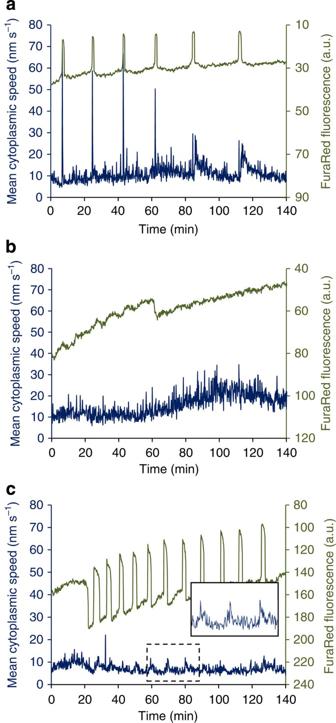Figure 3: Cytoplasmic speed peaks depend on free Ca2+oscillations. Peaks of mean cytoplasmic speed (blue) and free Ca2+levels (green) in a representative fertilized egg (a), fertilized egg treated with BAPTA-AM (b) and egg activated with SrCl2(c). When eggs were activated with SrCl2, Ca2+transients were not accompanied by even small speed peaks (insert in (c)). In all graphs, the increase in Ca2+level was reflected by a decrease in the intensity of FuraRed fluorescence. A peak in (b) was due to a shift in focus. Figure 3: Cytoplasmic speed peaks depend on free Ca 2+ oscillations. Peaks of mean cytoplasmic speed (blue) and free Ca 2+ levels (green) in a representative fertilized egg ( a ), fertilized egg treated with BAPTA-AM ( b ) and egg activated with SrCl 2 ( c ). When eggs were activated with SrCl 2 , Ca 2+ transients were not accompanied by even small speed peaks (insert in ( c )). In all graphs, the increase in Ca 2+ level was reflected by a decrease in the intensity of FuraRed fluorescence. A peak in ( b ) was due to a shift in focus. Full size image To determine whether Ca 2+ oscillations are essential for cytoplasmic movements, we recorded motion in 21 fertilized eggs loaded with the Ca 2+ chelator BAPTA, known to inhibit calcium oscillations without changing the basal level of intracellular Ca 2+ (ref. 32 ). This treatment suppressed high-amplitude speed peaks but elevated the mean basal cytoplasmic speed to 1.7-fold more than controls ( Fig. 3b ). Although BAPTA disrupted microtubules ( Supplementary Fig. S4 ), as observed in other systems [33] , [34] , this was unlikely to be responsible for the loss of speed peaks because specific disruption of microtubules did not cause a similar phenotype (see above). Interestingly, when we activated mouse eggs ( n =47) using SrCl 2, thus causing Ca 2+ oscillations similar to those seen after fertilization, only 30% (133/444) of Ca 2+ transients were accompanied by speed peaks. Moreover, these did not resemble the speed peaks of zygotes as they had very low amplitudes ( Fig. 3c ; Tables 1 and 3 ) and also were often delayed by 10–30 s with respect to the peak of the Ca 2+ transient. After-movements were present with 76.8% (341/444) of these Sr-induced Ca 2+ transients, but their amplitudes were also lower than in zygotes ( Tables 1 and 3 ). This suggests that although Ca 2+ oscillations are necessary for the rapid cytoplasmic movements, they are not sufficient to trigger distinct high-amplitude speed peaks. Thus, fertilization leads to further events that fully enable these motions. Table 3 Mean amplitudes of speed peaks and after-movements in embryos obtained by ICSI or by activation with SrCl 2 . Full size table Functional sperm proteins initiate cytoplasmic movements To further characterize the relative contribution made by either the sperm per se or the FC on both cytoplasmic speed peaks and Ca 2+ oscillations, we injected sperm directly into the egg, either immediately under the cortex or into the centre of the cell. Because formation of the FC depends on interplay between sperm chromatin and cortical actin and is distance-dependent [35] , FCs were only formed in the former group of injected eggs. In both cases, the injected sperm resulted in Ca 2+ oscillations and egg activation. However, whereas in eggs that formed FCs, 97% (101/104) of Ca 2+ transients were accompanied by speed peaks ( n =17 eggs, Fig. 4a ), in eggs without FCs, 71% (207/290) of Ca 2+ transients had speed peaks ( n =35 eggs; Fig. 4b ). Importantly, the mean amplitude of speed peaks was significantly lower in eggs without FCs, whereas in eggs with FCs amplitudes were similar to those in naturally fertilized ones ( Fig. 4a,b ; Tables 1 and 3 ). However, the mean amplitude of speed peaks during pronuclei formation and of the after-movements from all stages were similar in both groups ( Table 3 ), suggesting that mechanism of these particular movements may be FC-independent. 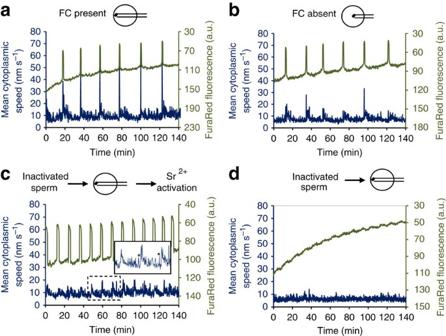Figure 4: High amplitude cytoplasmic speed peaks depend on the presence of the FC. Mean cytoplasmic speed (blue) and free Ca2+levels (green) in representative eggs subjected to ICSI. A fresh sperm head was injected under the cortex (a) or in the central part of the cytoplasm (b). A heat-inactivated sperm head was injected under the cortex and then the egg was either activated (c) or not activated (d) with SrCl2. In eggs injected with heated sperm heads and activated with SrCl2, small speed peaks were frequently present (insert in (c)). In all graphs, the increase in Ca2+level was reflected by a decrease in the intensity of FuraRed fluorescence. Figure 4: High amplitude cytoplasmic speed peaks depend on the presence of the FC. Mean cytoplasmic speed (blue) and free Ca 2+ levels (green) in representative eggs subjected to ICSI. A fresh sperm head was injected under the cortex ( a ) or in the central part of the cytoplasm ( b ). A heat-inactivated sperm head was injected under the cortex and then the egg was either activated ( c ) or not activated ( d ) with SrCl 2 . In eggs injected with heated sperm heads and activated with SrCl 2 , small speed peaks were frequently present (insert in ( c )). In all graphs, the increase in Ca 2+ level was reflected by a decrease in the intensity of FuraRed fluorescence. Full size image To further dissect the contribution of FCs to the triggering of cytoplasmic movements, we examined whether speed peaks would occur in response to injection of heat-inactivated sperm heads that are devoid of all functional proteins and serve as a source of DNA. Association of chromatin with the cortex is known to be sufficient to trigger FC-like formation [35] . Consequently, when heat-inactivated sperm heads were injected into the cortex and eggs activated by Sr 2+ , both Ca 2+ oscillations and FC formation were observed. In such zygotes ( n =25), 60.8% (48/79) of Ca 2+ transients were accompanied by speed peaks when the FCs were present (Stage 2). However, speed peak amplitudes remained relatively low ( Fig. 4c ; Table 3 ). Interestingly, the FC pulsations were also much less pronounced than those observed in normal zygotes and neither speed peaks nor FC pulsations were perfectly synchronized with the peaks of Ca 2+ transients but occurred 10–30 s later. No Ca 2+ oscillations were recorded in eggs injected with inactivated sperm and left without parthenogenetic activation ( Fig. 4d ). Together, these results suggest that high-amplitude speed peaks are associated with FC pulsations and are facilitated by functional proteins of the sperm. Cytoplasmic movements allow prediction of embryo viability Because we found that cytoplasmic movements correspond to the pattern of Ca 2+ oscillations and the quality of the cytoskeleton, we wondered whether the analysis of such movements might be predictive of developmental success. To address this, we fertilized 71 eggs in vitro , recorded their cytoplasmic movements throughout the period that FCs were present and then cultured embryos for 4 days. In the first instance, we related the pattern of cytoplasmic movements in each embryo with the total number of cells at this time ( Fig. 5a,b ). This showed that for different values of the mean interval between speed peaks, there were statistically significant linear and quadratic effects between the mean basal speed ( P =0.0005 and 0.0001 respectively, according to the negative binomial regression model) and the cell count in an embryo (on the log scale; Fig. 5c ). The mean cell count at the fourth day of development increased with the mean basal speed (up to 1.7 standard deviations (s.d.=6.7 nm s −1 ) away from the average of 12.2 nm s −1 of the mean basal speed values) after which it flattened off or declined ( Fig. 5c ). Moreover, for different values of the mean basal speed or its square, the mean number of cells after 4 days of development increased in proportion to the mean interval between speed peaks (1.3 times higher (95% CI: 1.07–1.47) for every 1 s.d., that is, ~7 min; P =0.0045, according to the negative binomial regression model, Fig. 5d ). Similar findings were observed when we examined developmental success by assessing the probability of development to the blastocyst stage ( Supplementary Fig. S5 ). This analysis suggests a linear relationship between the mean basal speed ( P =0.009, logistic regression model) and the logarithm of odds that the embryo achieves the blastocyst stage after 4 days of development: the probability of developing to a blastocyst increases as the mean basal speed increases. Moreover, we found that for every 1 s.d. increase in the mean interval between speed peaks the odds of an embryo developing into a blastocyst increased 2.3-fold (95% CI: 1.10–4.89; P =0.027, logistic regression model, Supplementary Fig. S5 ). 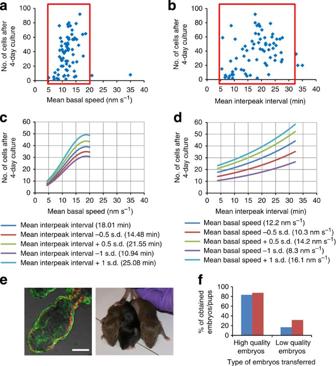Figure 5: Cytoplasmic movements as an indicator for viability of embryos. Correlation between mean basal speeds (a) or mean inter-speed peak intervals (b) recorded in zygotes and the number of cells in the embryos after 4 days of culture. (c) Mathematical model fitted to the data in (a), showing linear and quadratic correlation between mean basal speeds and number of cells in the 4-day-old embryos with an adjustment for different values of the mean interpeak intervals. (d) Mathematical model fitted to the data in (b), showing linear correlation between mean interpeak intervals and number of cells in the 4-day-old embryos with an adjustment for different values of the mean basal speeds. Graphic representation of the models in (c) and (d) was prepared for values in range indicated with red brackets in (a) and (b), respectively. (e) An egg cylinder (left) and 2-week-old pups (right) obtained from embryos scored as of high quality based on our model. Actin-labelled with phalloidin in green and Gata4 marking visceral endoderm in red. Scale bar 50 μm. (f) Efficiency of embryo transfers. Embryos were scored as of 'high quality' or 'low quality', according to our model, transferred at 2-cell stage to the recipient females and dissected at 6.5 (blue columns) or 19.5 dpc (red columns). Figure 5: Cytoplasmic movements as an indicator for viability of embryos. Correlation between mean basal speeds ( a ) or mean inter-speed peak intervals ( b ) recorded in zygotes and the number of cells in the embryos after 4 days of culture. ( c ) Mathematical model fitted to the data in ( a ), showing linear and quadratic correlation between mean basal speeds and number of cells in the 4-day-old embryos with an adjustment for different values of the mean interpeak intervals. ( d ) Mathematical model fitted to the data in ( b ), showing linear correlation between mean interpeak intervals and number of cells in the 4-day-old embryos with an adjustment for different values of the mean basal speeds. Graphic representation of the models in ( c ) and ( d ) was prepared for values in range indicated with red brackets in ( a ) and ( b ), respectively. ( e ) An egg cylinder (left) and 2-week-old pups (right) obtained from embryos scored as of high quality based on our model. Actin-labelled with phalloidin in green and Gata4 marking visceral endoderm in red. Scale bar 50 μm. ( f ) Efficiency of embryo transfers. Embryos were scored as of 'high quality' or 'low quality', according to our model, transferred at 2-cell stage to the recipient females and dissected at 6.5 (blue columns) or 19.5 dpc (red columns). Full size image To eliminate the possibility that our method of recording cytoplasmic movements caused any photodamage and to examine whether any possible light sensitivity depended on the post-fertilization stage of imaging, we compared development of zygotes that formed pronuclei at different times after the onset of recording. We found no evidence of any differences either between the mean cell numbers or the distribution of developmental stages achieved ( P >0.46, according to Student t -test, for any two compared groups and P =0.97, according to χ 2 test, respectively, Supplementary Fig. S5 ). We also compared development of imaged ( n =71) and non-imaged ( n =46) embryos ensuring that both groups were treated in the same way. No evidence for any differences in the mean number of cells or the distribution of embryos with different cell numbers between both groups was found ( P =0.75, according to Student t -test, and 0.19, according to χ 2 test, respectively; Supplementary Fig. S5 ). Finally, as the above results indicated that the pattern of cytoplasmic movements is predictive of pre-implantation development quality, we wished to determine whether these patterns of movements could predict which eggs would successfully develop to term. To this end, we imaged and analysed in vitro fertilized eggs and then grouped them accordingly to whether their cytoplasmic motion patterns would indicate good or poor developmental potential. Embryos with good potential were predicted to have after 4 days of culture between 25 and 52 (an average of 32) cells per embryo and to achieve the blastocyst stage in between 25 and 90% of cases (an average of 46.5%). Embryos classified as low quality would be predicted after 4 days to have between 9 and 24 cells (an average of 17), and that between 0 and 25% of them, an average of 10.7%, would achieve the blastocyst stage. The two groups of embryos were transferred at the two-cell stage to the recipient females. Those embryos scored as 'high quality' developed to the egg cylinder stage (6.5 dpc) 5 times more often (83.3%, 5/6 versus 16.7%, 1/6) and to full term (19.5 dpc) almost 3 times more often (2.77 times, 87.5%, 21/24 versus 31.6%, 6/19) than embryos scored as 'low quality' ( Fig. 5e,f ; Supplementary Table S3 ). Taken together, these findings indicate that post-fertilization cytoplasmic movements are predictive of developmental success and our method of imaging does not hinder embryo development. Non-invasive rapid time-lapse imaging combined with PIV analysis of cytoplasmic events after fertilization described here shows that sperm entry into the mouse egg triggers a series of unexpected rhythmic actomyosin contractions associated with cytoplasmic movements. At their maximum speed, these cytoplasmic movements have vectors directed towards the protrusion formed above the site of sperm entry that undergoes pulsations in synchrony with them. The speed peaks of the cytoplasmic movements correspond in timing with fertilization induced Ca 2+ transients, and they depend on calcium oscillations. Finally, we show that analysis of the interval between peaks provides a novel non-invasive and very rapid way of assessing the vitality of the embryo and its ability to succeed in development. The involvement of the actomyosin cytoskeleton in mediating cytoplasmic movements is evident from our findings that inhibition of MLCK or treatments that either stabilized or depolymerized F-actin diminished both speed peaks and the basal cytoplasmic speed. The movements also depend on Ca 2+ transients, because they were prevented by chelating Ca 2+ with BAPTA. One possibility is that Ca 2+ -dependent kinases such as Ca 2+ /calmodulin-dependent kinase II or conventional protein kinase C participate in triggering the movements as these enzymes are known both to regulate the cytoskeleton [11] and respond to Ca 2+ oscillations [36] , [37] , [38] . However, whereas the amplitude of Ca 2+ oscillations are similar throughout the whole post-fertilization period (except for the first Ca 2+ spike that is usually bigger than subsequent ones [31] ), the amplitude of the speed peaks increases at onset of FC formation and decreases on FC regression. Moreover, the Ca 2+ transients evoked by parthenogenetic activation are not sufficient to promote fast, oscillatory cytoplasmic movements suggesting that further fertilization-associated factors must enable the movements to take place. The coincidence of speed peaks with actomyosin-mediated rhythmic movements of the FC suggests that these are manifestations of the same process. This is further borne out by studies of FC formation after sperm injection. As FC formation requires interaction of chromatin with cortical proteins [35] , it does not occur when sperm is injected deep into the egg. Accordingly, eggs fertilized in this way showed much weaker speed peaks than in zygotes with FCs. The fact that speed peaks, although weak, were still present, could be because sperm chromatin was positioned close enough to the cell surface to cause some reorganization of the cortical actomyosin. Although insufficient to produce a well-defined FC, this would still be able to enhance weak cytoplasmic movements. Alternatively, the speed peaks could be triggered by contractions of the cortical actomyosin accumulated above the maternally derived chromatin. Indeed, we frequently could see that a bulge formed above the set of maternal chromosomes pulsates in a way similar to the FC. It is also possible that low-amplitude speed peaks may be an effect of general contractility of the actomyosin cytoskeleton, not associated with the cortex. The last two possibilities could also explain why there are some low-amplitude speed peaks visible in the Sr 2+ -activated parhenogenotes. High-speed movements were also not triggered, and FC motions were very much diminished in Sr 2+ -activated eggs injected with heat-inactivated sperm heads. Thus, the sperm may well contribute proteins that facilitate FC motions and cytoplasmic movements that are inactivated by heat treatment. It is also possible that differences observed between normal zygotes and embryos injected with inactivated sperm followed by Sr 2+ activation may be due to the altered characteristics of the Ca 2+ transients themselves. The dynamics of typical Sr 2+ -induced Ca 2+ peaks differ from those of Ca 2+ peaks triggered by fertilization [39] , [40] . Moreover, frequency of the Sr 2+ -induced Ca 2+ oscillations was very high under our conditions, and this seemed to affect negatively generation of high-amplitude speed peaks. As the timing and pattern of cytoplasmic movements mirror these of Ca 2+ oscillations and depend on the integrity of the cytoskeleton, we find that they provide a powerful indicator of the embryo quality. Our data shows that embryos with low mean basal speed (below 10 nm s −1 ; indicates poor quality of the actomyosin cytoskeleton), as well as embryos with very frequent speed peaks (interpeak interval below 10 min; reflecting frequent Ca 2+ transients), rarely develop to the blastocyst stage in vitro or to full term in vivo . This result accords with findings that both functional actin cytoskeleton and correct pattern of Ca 2+ transients (especially the total time of Ca 2+ elevation) are crucial for development [13] , [17] , [18] , [41] , [42] , [43] . Unfortunately, these factors cannot be used in research and medical facilities to select good quality embryos as their assessment involves invasive procedures using fluorescent dyes and harmful irradiation. Thus, current practice in the in vitro fertilization clinic is to assess the viability of embryos on day 3 from their morphology and growth at day 5, because of unreliability of the 3-day assessment [44] , [45] , [46] . A considerable advance may be offered by imaging and monitoring of a series of parameters over the first two days of development [47] . Our present findings suggest that, in future, it might be possible to assess the vitality of the embryo and its ability to succeed in development by using non-invasive imaging over a much shorter period of time, just 2 h after the time of fertilization. In conclusion, we have identified the importance of the sperm in triggering a dynamic oscillatory behaviour of the actomyosin cytoskeleton at fertilization. The ensuing movements have a pattern and timing that provides a powerful method of assessing an egg's ability to achieve its full developmental potential. As such, our method has considerable potential in finding practical application in the assisted reproduction clinic. Animals Animals were maintained in the Animal Facility of Gurdon Institute at 12:12 light cycle and provided with food and water ad libitum . All experiments were conducted in compliance with the University of Cambridge regulations. Collection of eggs and sperm F1 (C57Bl6×CBA) mouse females were superovulated with intraperitoneal injection of 7.5 IU of pregnant mare serum gonadotrophin (PMSG, Intervet) followed 48 h later by 7.5 IU of human chorionic gonadotrophin (hCG, Intervet). Oocytes and zygotes were recovered 14–16 h later from oviducts. Parthenogenetic activation was performed by incubating eggs for 4 h in M2 medium without Ca 2+ /Mg 2+ supplemented with 10 mM SrCl 2 . Germinal vesicle oocytes were isolated from ovaries to M2 medium supplemented with 150 μg ml −1 dibutyryl cyclic AMP. Epididymal sperm was isolated from F1 males and capacitated in 0.5 ml of fertilization medium with 4 mg ml −1 bovine serum albumin (BSA) [48] . Embryos were cultured in KSOM medium. In some experiments, embryos were pre-incubated for 20 min with 30 μM BAPTA-AM (to chelate Ca 2+ ), 5 μg ml −1 nocodazole (to depolimerize microtubules), 2 μg ml −1 cytochalasin D (to depolimerize F-actin), 10 μM taxol (to stabilize microtubules), 100 nM jasplakinolide (to stabilize F-actin), or 25 μM ML-7 (to inhibit MLCK and therefore myosin II activation [49] ) and then transferred to pure KSOM (BAPTA-treated embryos) or to KSOM containing the respective drug (rest of the treated embryos). Incubations with ML-7 were done without a mineral oil overlay that would have absorbed ML-7. Drug concentrations were tested in preliminary studies and were shown to effectively inhibit extrusion of 2PB under our experimental conditions. Imaging and PIV analysis of cytoplasmic movements In most experiments, zygotes were imaged in a single plane under an inverted confocal microscope (Zeiss LSM 510 Meta) at 37.5 °C and 5% CO 2 . DIC images were captured every 10 s using a 633 nm HeNe laser. To measure free Ca 2+ ion concentration, embryos were pre-incubated for 20 min in 5 μM FuraRed-AM (Invitrogen) and FuraRed and DIC images were obtained simultaneously with a 488 nm argon laser. In experiments in which correlations between cytoplasmic movements and developmental potential of the embryos were examined, zygotes were imaged in a single plane in transmitted light under standard non-confocal microscopes (Zeiss Axiovert or Deltavision) every 10 s for 2.5 h. In experiments in which cytoplasmic movements in the cortex and central parts of zygotes were compared, embryos were imaged on the Deltavision microscope in 11 planes every 6 μm, every 10 s for 3 h. Optical specifications of all imaging systems used are summarized in Supplementary Table S4 . Intensity of FuraRed fluorescence was measured using ImageJ software. Images were analysed using custom written software in MATLAB (Mathworks) using algorithms adapted from MatPIV v1.6.1 (ref. 50 ). The algorithm was based on that used in PIV, a standard analysis technique used extensively in fluid dynamics [23] , [24] , [25] , [26] that involves cross-correlating image sub-regions between sequential pairs of images. In the PIV analysis, each image was divided into square interrogation regions and the cross-correlation coefficient distribution was calculated within a larger region in the next image in the sequence. The peak of the cross-correlation coefficient distribution gave the most likely location in the second image of the material in the interrogation region in the first image. This was then used to calculate the displacement vector over the time between images ( Fig. 1a ). As the displacement of the pattern of contrast of an area of pixels is being measured over many pixels, it is possible to accurately measure sub-pixel movements with this technique [24] , [26] , [51] . For more detailed description of the PIV method and its resolution, see Supplementary Methods . Analysis of cytoplasmic speed and movement direction In zygotes that displayed oscillatory changes in the cytoplasmic speed, the mean basal speed was measured in intervals between end of the after-movement and beginning of the subsequent speed peak or in a period after the last after-movement ( Fig. 1d ). For zygotes that did not display the speed oscillations, mean basal speed was calculated for whole recording period. In most cases, direction of the cytoplasmic movements was based on the mean vector of all the vectors produced by PIV in the zygote. In some zygotes, vectors formed a pair of vortices and then their common axis was taken as the direction. The direction of highly irregular vector patterns was visually assessed from the direction of the majority of high-magnitude vectors. Intracytoplasmic sperm injection ICSI was carried out using Leica micromanipulators and Leica inverted microscope. In some experiments, heat-inactivated sperm (30 min in 60 °C) was used instead of freshly isolated sperm. The sperm suspension was mixed with M2 medium containing 10% polyvinylpyrrolidone (Mr=360 kDa). Sperm were delivered into the oocytes' cytosol, using a piezo micropipette-driving unit (IntraCel PMAS-CT150, PrimeTech). In vitro fertilization and embryo transfers To examine a correlation between cytoplasmic movements and developmental potential of the embryos, 10 μl of capacitated sperm suspension was added to eggs surrounded by cumulus cells, and, then, gametes were co-incubated for 2 h. In experiments testing specificity of inhibitors or involving live imaging of actin and myosin, before fertilization, eggs were treated shortly with acidic Tyrode's solution (pH=2.5) to remove zonas, then were mixed with approximately 1 μl of capacitated sperm suspension and incubated together for 30 min. In both cases, fertilization was performed in fertilization medium supplemented with 4 mg ml −1 BSA [48] . Embryos at 2-cell stage were transfer to oviducts of recipient F1 females mated with vasectomised males on 0.5 dpc. They were dissected on 6.5 or 19.5 dpc. Live imaging of actin filaments and myosin II Constructs encoding actin-binding domain of utrophin fused to EGFP (UtrCH–EGFP [28] ), myosin II regulatory light chain fused to GFP (MyoRLC–GFP [29] ), and protein marker Gap43 tagged with RFP [52] were cloned into a pBluescript RN3P vector, and mRNA was synthesized from T3 promotor, using mMessage mMachine T3 kit (Ambion). mRNAs (pipette concentration 0.5 μg μl −1 for UtrCH–EGFP and MyoRLC–GFP and 0.36 μg μl −1 for Gap43–RFP) were injected into germinal vesicle oocytes that were subsequently cultured for approximately 5 h in M2 with 150 μg ml −1 dibutyryl cyclic AMP and then washed out and transferred to M16 medium to mature. Oocytes that 16 h later achieved metaphase of the 2nd meiotic division were selected for in vitro fertilization and then were imaged every 10–15 s on an inverted spinning disc confocal microscope (Zeiss). UtrCH–EGFP, MyoRLC–GFP and Gap43–RFP fluorescence intensities were measured in the FC cortex and in the cytoplasm using ImageJ software. Values obtained for cortical UtrCH–EGFP, MyoRLC–GFP and Gap43–RFP were standardized with respective intensities obtained for the cytoplasm to eliminate any intensity changes that were caused by imaging artefacts, for example, fluctuations in laser power. The final results were then presented as ratios between UtrCH–EGFP and Gap43–RFP or MyoRLC–GFP and Gap43–RFP standardized intensities to eliminate any intensity changes caused by shifts in focus. Immunostaining Embryos were fixed in 4% PFA and processed as described in Supplementary Methods . Statistical analysis Statistical analyses were performed ether using Student's t -test, χ 2 test or appropriate regression models. Because of the sequential nature of the experiments performed and the a priori nature of the questions that we sought to address, we assessed statistical significance at the 5% level. To determine relationships between mean basal speed or mean interval between speed peaks and the total number of cells produced after 4 days of development (that is, the four-day cell count), we fitted negative-binomial models to the cell counts of the embryos, with a logarithmic link function relating the mean cell count to the linear combination of explanatory variables: the mean basal speed, the square of mean basal speed, the mean interval between speed peaks, the square of the mean interval between speed peaks, and the various interactions between the basal speed and speed peaks variables. In our initial analysis, we took into account the potential confounding effects of the imaging system used (Zeiss or Deltavision) on embryo development. However, as we found that the interaction between the analysed parameters, the quadratic effect of the mean interval between speed peaks and the image system were not statistically significant and did not contribute any further explanatory power, we dropped them in our final analysis. The likelihood ratio test of the full model, with all the variables mentioned above, included in comparison with the final model, yielded a non-statistically significant change in the log-likelihood ( P =0.53). Negative-binomial modelling of the cell count was chosen over the more standard Poisson regression modelling of the cell count to account for extra-Poisson variation observed in the cell count data [53] . To investigate the relationship between the same explanatory variables as described above and the probability that a zygote develops into a blastocyst (that is, achieves at least 32-cell stage), we also analysed our data by fitting logistic regression models, after dichotomizing total number of cells produced after 4 days of development into a binary variable, indicating whether or not the total cell count exceeded 31 cells. The final logistic model included the same explanatory variables as those in the final negative-binomial model. (The likelihood ratio test of the full model against the final model yielded a non-statistically significant change in the log-likelihood ( P =0.30)). How to cite this article: Ajduk, A. et al . Rhythmic actomyosin-driven contractions induced by sperm entry predict mammalian embryo viability. Nat. Commun. 2:417 doi: 10.1038/ncomms1424 (2011).